Differential developmental requirement and peripheral regulation for dermal Vγ4 and Vγ6T17 cells in health and inflammation Dermal IL-17-producing γδT cells have a critical role in skin inflammation. However, their development and peripheral regulation have not been fully elucidated. Here we demonstrate that dermal γδT cells develop from the embryonic thymus and undergo homeostatic proliferation after birth with diversified TCR repertoire. Vγ6T cells are bona fide resident, but precursors of dermal Vγ4T cells may require extrathymic environment for imprinting skin-homing properties. Thymic Vγ6T cells are more competitive than Vγ4 for dermal γδT cell reconstitution and TCRδ −/− mice reconstituted with Vγ6 develop psoriasis-like inflammation after IMQ-application. Although both IL-23 and IL-1β promote Vγ4 and Vγ6 proliferation, Vγ4 are the main source of IL-17 production that requires IL-1 signalling. Mice with deficiency of IL-1RI signalling have significantly decreased skin inflammation. These studies reveal a differential developmental requirement and peripheral regulation for dermal Vγ6 and Vγ4 γδT cells, implying a new mechanism that may be involved in skin inflammation. The skin has a unique composition of immune cells. In addition to adaptive αβT cells, many innate immune cells including dermal dendritic cells and γδT cells reside in the skin to establish a skin immune network that has a critical role in host defence and tissue repair [1] . In mice, Vγ5Vδ1T cells, named dendritic epidermal T cells (DETCs), uniquely reside in the epidermis during fetal development [2] . These cells have been shown to recognize a putative antigen (Ag) expressed on the keratinocytes (KCs) and are involved in the skin immunosurveillance [3] . Recently, a new subset of γδT cells has been identified in the skin [4] , [5] , [6] . In comparison with DETCs, this subset of γδT cells resides mainly in the dermis under the steady condition. They bear different Vγ usage and are the major interleukin (IL)-17 producers in the skin upon IL-23 or toll-like receptor-7/8 agonist imiquimod (IMQ) stimulation [4] , [7] , [8] . However, their development, trafficking and peripheral regulation are not fully understood. Previous studies have shown that DETCs are derived from early fetal thymic precursor cells [9] . DETCs are home to the skin between embryonic days 16 and 18 before birth. In addition, IL-17-producing γδT (γδT17) cells in the periphery such as lymph nodes (LN) also develop in the thymus after birth through a transforming growth factor-β-dependent mechanism [10] . It appears that different subsets of γδT17 cells migrate from the thymus into the periphery in a functional wave manner [11] . At the molecular level, a thymic epithelial cell determinant, Skint-1, has a critical role in the development of interferon (IFN)-γ-producing versus IL-17-producing γδT cells [12] . Transcriptional factor Sox13 is essential for all IL-17-committed Vγ4 T-cell development and function including dermal Vγ4 T cells [13] , [14] . Previous studies have also identified that scavenger receptor SCART2 is uniquely expressed in IL-17-producing γδT cells homing to the peripheral LN and dermis [15] . Furthermore, studies have shown that γδT cells can traffick between LN and skin [13] , [16] , posing the question whether dermal γδT17 cells develop similarly as other peripheral γδT cells. Through bone marrow (BM) chimeras where BM cells were transplanted into lethally irradiated host mice, it showed that 90% of dermal γδT cells were from host origin, whereas ∼ 10% of dermal γδT cells were from donor BM [6] , suggesting that BM cells may contain precursor cells that give rise to dermal γδT cells. Although early studies from Gray et al . [5] suggested that dermal γδT cells could not be reconstituted by BM cells , their later studies showed that IL-17-producing Vγ4 T cells could be reconstituted by BM [13] . However, a recent study demonstrated that IL-17-producing γδT cells develop before birth and maintain in adult mice as self-renewing cells [11] , thus leaving the role of BM in the generation of dermal γδT cells uncertain. Furthermore, the detailed information for mature dermal γδT cell migration into skin is lacking. Previous studies have shown that embryonic trafficking of DETCs to skin requires E/P selectin ligands and CCR4 (ref. 17 ). CCR10 also has a critical role in the migration and location of DETCs [18] , [19] . When and where dermal γδT cells develop and migrate into the skin are poorly understood. Here we demonstrate that dermal γδT cells developed from fetal thymus and undergo homeostatic proliferation after birth, with diversified TCR repertoire. IL-17-producing Vγ6 T cells are bona fide resident in dermis and are reconstituted from fetal thymus, whereas thymic Vγ4 T cells may require extrathymic environment for imprinting of their skin-homing properties. Chemokine receptor CCR6 is critical for dermal Vγ4 but not for Vγ6 T-cell migration. It appears that thymic Vγ6 T cells are more competitive than Vγ4 for dermal γδT cell reconstitution. In addition, Vγ6 T cells are pathogenic and can induce skin inflammation, whereas Vγ4 T cells are preferentially expanded and are the major IL-17 producers in the IMQ model of psoriasis-like skin inflammation. Although IL-23 and IL-1β are capable of driving dermal Vγ4 and Vγ6 T-cell proliferation, IL-17 is mainly produced by Vγ4, for which IL-1 signalling is essential. Deficiency of IL-1 receptor (IL-1R) signalling pathway significantly decreases both IL-23 and IMQ-induced skin inflammation. These results demonstrate the importance of IL-1β in the regulation of the proliferation and IL-17 production by different subsets of dermal γδT cells when interplaying with IL-23, implying a new mechanism that may be involved in skin inflammation. Dermal γδT cell development in mice before and after birth To investigate the development of dermal γδT cells, skin tissues from embryonic or neonatal pups were used to track dermal γδT cell appearance. γδTCR hi epidermal γδT cells were readily seen on E20 and day 1 ( Supplementary Fig. 1a and Fig. 1a ), consistent with a previous report [9] . In contrast, γδTCR int dermal γδT cells were scarce on E20 or day 1. Dermal γδT cells became obvious on day 3 and had similar frequency as adult mice on day 14 ( Fig. 1a ). Next we examined the TCR repertoire of developing dermal γδT cells. TCR repertoire of dermal γδT cells on days 3–5 showed almost exclusive Vγ6 ( Fig. 1b ). Dermal Vγ4 became apparent on day 7. In adult mice, dermal γδT cells expressed TCRs mainly containing Vγ6 and Vγ4 ( Fig. 1b ). In contrast, TCR repertoire of thymic γδT cells on days 1–3 showed that Vγ1, Vγ4 and Vγ6 while Vγ6 was gradually decreased over the time ( Fig. 1b ). Side-by-side comparison studies indicated that Vγ1 and Vγ4 were the predominant γδT cells in the BM. Ki-67 staining suggested that both dermal Vγ6 and Vγ4 T cells had a significant more homeostatic proliferation at early days and then maintained lower proliferation rate in adult mice ( Fig. 1c ). In addition, dermal γδT cells were capable of producing IL-17 ( Fig. 1d ). We also examined γδT cells in the lung. Lung γδT cells were apparent on E20 and contained both Vγ6 and Vγ4. In contrast to dermal γδT cells, Vγ6 T cells were more than Vγ4 in the lung even after birth and in adult mice ( Supplementary Fig. 1b ). Taken together, these results suggest that dermal γδT cells migrate into the skin before birth and are further expanded after birth with more diversified TCR repertoire. 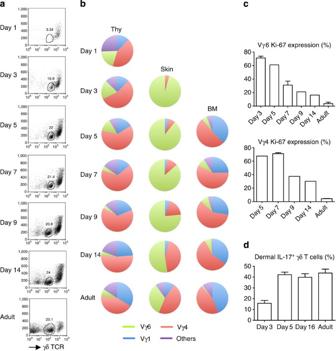Figure 1: Development of dermal γδT cells. (a) Whole-skin cell suspensions prepared from C57Bl/6 WT mice at different days (n=3–5) after birth were stained with CD3 and γδTCR, and the frequency of γδTCRintdermal γδT cells was analysed by flow cytometry. Flow plots gated on CD3+cells are representative of three independent experiments with similar results. (b) Thymocytes (Thy), whole-skin cells and BM cells from different days after birth were stained with CD3, γδTCR and Vγ (Vγ 1, 4, 6) mAbs. Percentages of Vγ1, Vγ4 and Vγ6 γδT cells were analysed by flow cytometry and summarized in pie chart. (c) Percentages of Ki-67 expression on dermal Vγ4 and Vγ6 T cells were analysed by flow cytometry. Cells were gated on CD3intγδTCRintVγ4+or Vγ6+cells. Data are shown as mean±s.e.m. (d) Whole-skin cells were stimulated with phorbol myristate acetate (PMA) plus ionomycin for 5 h, and the percentage of IL-17-producing γδT cells gated on CD3intγδTCRintcells was analysed by flow cytometry. Data are shown as mean±s.e.m. Figure 1: Development of dermal γδT cells. ( a ) Whole-skin cell suspensions prepared from C57Bl/6 WT mice at different days ( n =3–5) after birth were stained with CD3 and γδTCR, and the frequency of γδTCR int dermal γδT cells was analysed by flow cytometry. Flow plots gated on CD3 + cells are representative of three independent experiments with similar results. ( b ) Thymocytes (Thy), whole-skin cells and BM cells from different days after birth were stained with CD3, γδTCR and Vγ (Vγ 1, 4, 6) mAbs. Percentages of Vγ1, Vγ4 and Vγ6 γδT cells were analysed by flow cytometry and summarized in pie chart. ( c ) Percentages of Ki-67 expression on dermal Vγ4 and Vγ6 T cells were analysed by flow cytometry. Cells were gated on CD3 int γδTCR int Vγ4 + or Vγ6 + cells. Data are shown as mean±s.e.m. ( d ) Whole-skin cells were stimulated with phorbol myristate acetate (PMA) plus ionomycin for 5 h, and the percentage of IL-17-producing γδT cells gated on CD3 int γδTCR int cells was analysed by flow cytometry. Data are shown as mean±s.e.m. Full size image Fetal thymus is required for dermal γδT cell development We next examined if development of dermal γδT cells was confined to the fetal thymus. To this end, we transplanted BM cells or BM cells plus neonatal thymocytes from wild-type (WT) C57Bl/6 mice (CD45.2) into CD45.1 congenic SJL mice. Mice transplanted with BM cells alone had significantly lower dermal γδT cells as compared with mice transplanted with BM plus neonatal thymocytes ( Fig. 2a ). In mice transplanted with BM alone, the majority of CCR6 + dermal γδT cells were host resident, whereas ∼ 15% were donor origin. Dermal γδT cells from both sources were capable of secreting IL-17 ( Fig. 2b ). In contrast, mice were transplanted with BM plus neonatal thymocytes, almost all dermal γδT cells were of donor origin ( Fig. 2b ). To further confirm that BM cells contain precursors of dermal γδT cells, TCRδ-deficient mice were used as host to receive BM cells from SJL mice. Indeed, dermal γδT cells could be reconstituted from donor BM and were able to secrete IL-17 ( Fig. 2c ). To determine whether the thymus is required for dermal γδT cell development, we examined dermal γδT cells in athymic nude mice. As shown in Supplementary Fig. 2 , dermal γδT cells were lacking in nude mouse skin. In addition, γδT cells in BM were also scarce. We then transplanted BM cells from CD45.1 SJL mice into CD45.2 nude or WT mice. Consistent with Fig. 2a , dermal γδT cells were reconstituted in both WT and nude mice, and these cells were able to secrete IL-17 ( Fig. 2d ). Dermal γδT cells were significantly expanded in nude mice, compared with those in WT recipients ( Fig. 2d ). Further TCR usage analysis indicated that Vγ4 and Vγ1 were predominant in WT mice, whereas nude mice reconstituted with WT BM had exclusively Vγ4. No Vγ6 was observed ( Fig. 2d ). 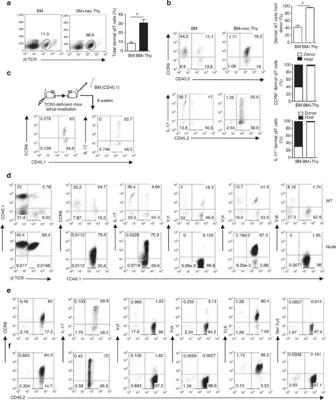Figure 2: Fetal thymus is required for dermal γδT cell development and Vγ6 T cell reconstitution while dermal Vγ4 T cells originate mainly from BM. BM cells or BM cells plus neonatal thymocytes (BM+neo Thy) from C57Bl/6 WT mice (CD45.2) were transplanted into lethally irradiated SJL mice (CD45.1,n=4–5). (a) Eight weeks after reconstitution, percentage of dermal γδT cells gated on CD3+cells from recipient mice was analysed by flow cytometry, and total frequency of dermal γδT cells was summarized. Data are shown as mean±s.e.m. *P<0.05 (unpaired Student’st-test). (b) Whole-skin cells were stimulated with PMA plus ionomycin for 5 h. CCR6+and IL-17+CD3intγδTCRintcells were analysed by flow cytometry. Flow plots were gated on CD3intγδTCRintcells. Percentages of dermal γδT cells from donor are shown as mean±s.e.m. *P<0.05 (unpaired Student’st-test). Degree of chimerism of CCR6+and IL-17-producing dermal γδT cells are also shown as open bars (donor) and filled bars (host). Data are representative of at least three independent experiments with similar results. (c) BM cells from SJL mice (CD45.1) were transplanted into lethally irradiated TCRδ KO mice (CD45.2). After 8 weeks of reconstitution, CCR6+and IL-17-producing dermal γδT cells were analysed by flow cytometry. Flow plots gated on CD3+γδTCR+cells are representative of two independent experiments with similar results. (d) BM cells from SJL mice (CD45.1) were transplanted into lethally irradiated C57Bl/6 WT mice or nude mice (CD45.2). After 8 weeks of reconstitution, percentage of dermal γδT cells gated on CD3+cells was detected by flow cytometry. Furthermore, CCR6 expression and Vγ usage (Vγ1, 4, 6) of dermal γδ T cells and intracellular IL-17 by dermal γδT cells after PMA plus ionomycin stimulation were also analysed by flow cytometry. Flow plots were gated on CD3intγδTCRintcells. (e,f) Thymocytes from C57Bl/6 WT neonatal (e) or E18 (f) pups plus BM cells from TCRδ KO mice were transplanted into lethally irradiated SJL mice. After 8 weeks of reconstitution, CCR6 expression and Vγ usage (Vγ1, 4, 6) of dermal γδT cells and intracellular IL-17 after PMA plus ionomycin stimulation were analysed by flow cytometry. Flow plots were gated on CD3intγδTCRintcells. Figure 2: Fetal thymus is required for dermal γδT cell development and Vγ6 T cell reconstitution while dermal Vγ4 T cells originate mainly from BM. BM cells or BM cells plus neonatal thymocytes (BM+neo Thy) from C57Bl/6 WT mice (CD45.2) were transplanted into lethally irradiated SJL mice (CD45.1, n =4–5). ( a ) Eight weeks after reconstitution, percentage of dermal γδT cells gated on CD3 + cells from recipient mice was analysed by flow cytometry, and total frequency of dermal γδT cells was summarized. Data are shown as mean±s.e.m. * P <0.05 (unpaired Student’s t -test). ( b ) Whole-skin cells were stimulated with PMA plus ionomycin for 5 h. CCR6 + and IL-17 + CD3 int γδTCR int cells were analysed by flow cytometry. Flow plots were gated on CD3 int γδTCR int cells. Percentages of dermal γδT cells from donor are shown as mean±s.e.m. * P <0.05 (unpaired Student’s t -test). Degree of chimerism of CCR6 + and IL-17-producing dermal γδT cells are also shown as open bars (donor) and filled bars (host). Data are representative of at least three independent experiments with similar results. ( c ) BM cells from SJL mice (CD45.1) were transplanted into lethally irradiated TCRδ KO mice (CD45.2). After 8 weeks of reconstitution, CCR6 + and IL-17-producing dermal γδT cells were analysed by flow cytometry. Flow plots gated on CD3 + γδTCR + cells are representative of two independent experiments with similar results. ( d ) BM cells from SJL mice (CD45.1) were transplanted into lethally irradiated C57Bl/6 WT mice or nude mice (CD45.2). After 8 weeks of reconstitution, percentage of dermal γδT cells gated on CD3 + cells was detected by flow cytometry. Furthermore, CCR6 expression and Vγ usage (Vγ1, 4, 6) of dermal γδ T cells and intracellular IL-17 by dermal γδT cells after PMA plus ionomycin stimulation were also analysed by flow cytometry. Flow plots were gated on CD3 int γδTCR int cells. ( e , f ) Thymocytes from C57Bl/6 WT neonatal ( e ) or E18 ( f ) pups plus BM cells from TCRδ KO mice were transplanted into lethally irradiated SJL mice. After 8 weeks of reconstitution, CCR6 expression and Vγ usage (Vγ1, 4, 6) of dermal γδT cells and intracellular IL-17 after PMA plus ionomycin stimulation were analysed by flow cytometry. Flow plots were gated on CD3 int γδTCR int cells. Full size image Since dermal γδT cells consist both Vγ4 and Vγ6 TCR repertoire in adult mice, we reasoned whether dermal Vγ6 T cells were from fetal thymus. To exclude precursors of dermal γδT cells from BM, BM cells from TCRδ-deficient mice were mixed with neonatal thymocytes ( Fig. 2e ). Dermal γδT cells were almost all donor origin and predominately expressed Vγ6. Since previous study showed that IL-17-producing γδT cells develop from embryonic thymus [11] , we further used E18 embryonic thymocytes for reconstitution. Similar as neonatal thymocytes, dermal γδT cells from E18 thymocytes showed exclusively donor origin and were capable of producing IL-17 and predominantly expressed Vγ6 ( Fig. 2f ). These data suggest that IL-17-producing dermal γδT cells can be reconstituted from both fetal thymus and adult BM with different TCR repertoire, and thymus is absolutely required for dermal γδT cell development. Thymic Vγ4 requires extrathymic environment for skin homing E18 and neonatal thymocytes contain both Vγ4- and Vγ6-expressing γδT cells with similar frequency ( Fig. 1b ). However, mice transplanted with E18 or fetal thymocytes had exclusive Vγ6 T-cell reconstitution, whereas majority of Vγ4 T cells were reconstituted from BM ( Fig. 2 ). To further validate this, we sorted Vγ4 or Vγ6 T cells from neonatal thymocytes (CD45.2) and mixed with BM cells (CD45.1) as a source of BM Vγ4. TCRδ-deficient mice were used as recipient mice. The ratio of Vγ4 from both sources was approximately at 1:1 as well as Vγ6 to Vγ4 ( Fig. 3a ). As shown in Fig. 3b , mice transplanted with Vγ4 from neonatal thymus plus BM cells had dermal γδT cells expressing Vγ4, predominately from BM (>80%). In contrast, mice transplanted with neonatal Vγ6 plus BM cells had dermal γδT cells expressing Vγ6, exclusively from neonatal thymus ( Fig. 3b ). Both Vγ4 and Vγ6 T cells were capable of secreting IL-17 ( Fig. 3b ). These data suggest that Vγ4 and Vγ6 dermal γδT cells may have a differential developmental requirement. 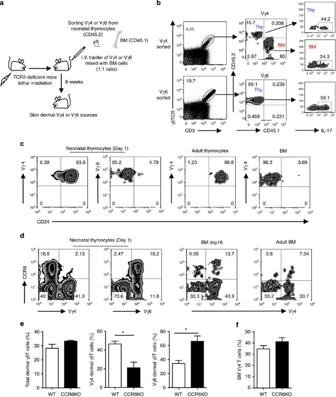Figure 3: Thymic Vγ4 T cells require extrathymic environment for imprinting of skin-homing properties. (a,b) Sorted Vγ4 or Vγ6 neonatal thymocytes (Thy) from C57Bl/6 WT mice (CD45.2) mixed with BM cells from SJL mice (CD45.1) were transferred into lethally irradiated TCRδ KO mice (n=3–5). The ratio of Vγ4 from both sources was around 1:1 as well as Vγ6 to Vγ4 (based on Vγ4 frequency in BM). After 8 weeks of reconstitution, total dermal γδT cells (a) and the sources of Vγ4 or Vγ6T cells as well as intracellular IL-17 stimulated with PMA plus ionomycin (b) were determined by flow cytometry. Flow plots were gated on CD3+γδTCR+cells. (c,d) CD24 (c) and CCR6 (d) expression by Vγ4 or Vγ6 cells on neonatal Thy, adult Thy, BM cells (Day16) and adult BM cells were determined by flow cytometry. Flow plot gated on CD3+γδTCR+cells are representative of three independent experiments with similar results. (e,f) Whole-skin cells (e) or BM cells (f) from C57Bl/6 WT mice or CCR6KO mice (n=3) were stained with CD3, γδTCR, Vγ4 and Vγ6. Percentages of total dermal γδT cells as well as dermal Vγ4 and Vγ6 cells or BM Vγ4 cells were analysed by flow cytometry. Data are shown as mean±s.e.m. and are representative of three independent experiments with similar results. *P<0.05 (unpaired Student’st-test). Figure 3: Thymic Vγ4 T cells require extrathymic environment for imprinting of skin-homing properties. ( a , b ) Sorted Vγ4 or Vγ6 neonatal thymocytes (Thy) from C57Bl/6 WT mice (CD45.2) mixed with BM cells from SJL mice (CD45.1) were transferred into lethally irradiated TCRδ KO mice ( n =3–5). The ratio of Vγ4 from both sources was around 1:1 as well as Vγ6 to Vγ4 (based on Vγ4 frequency in BM). After 8 weeks of reconstitution, total dermal γδT cells ( a ) and the sources of Vγ4 or Vγ6T cells as well as intracellular IL-17 stimulated with PMA plus ionomycin ( b ) were determined by flow cytometry. Flow plots were gated on CD3 + γδTCR + cells. ( c , d ) CD24 ( c ) and CCR6 ( d ) expression by Vγ4 or Vγ6 cells on neonatal Thy, adult Thy, BM cells (Day16) and adult BM cells were determined by flow cytometry. Flow plot gated on CD3 + γδTCR + cells are representative of three independent experiments with similar results. ( e , f ) Whole-skin cells ( e ) or BM cells ( f ) from C57Bl/6 WT mice or CCR6KO mice ( n =3) were stained with CD3, γδTCR, Vγ4 and Vγ6. Percentages of total dermal γδT cells as well as dermal Vγ4 and Vγ6 cells or BM Vγ4 cells were analysed by flow cytometry. Data are shown as mean±s.e.m. and are representative of three independent experiments with similar results. * P <0.05 (unpaired Student’s t -test). Full size image To gain insight into this difference, we examined maturation status of Vγ4 and Vγ6 T cells in thymus and BM. As shown in Fig. 3c , almost all Vγ6 T cells in neonatal thymus had mature phenotype (CD24 lo ). In contrast, most Vγ4 T cells were immature (CD24 hi ) in neonatal or adult thymus. This was consistent with CD44 CD62L staining patterns where the majority of Vγ6 T cells in E20 or neonatal stage were CD44 hi CD62L lo while most Vγ4 T cells were CD44 lo ( Supplementary Fig. 3a ). Strikingly, Vγ4 T cells from BM were almost all mature (CD24 lo ) ( Fig. 3c ), suggesting that Vγ4 T cells may require extrathymic environment for maturation. To rule out the possibility that Vγ4 T cells may have delayed maturation in the thymus as previously reported [13] , we used thymocytes from different ages of mice ranging from days 2 to 17 for dermal γδT reconstitution studies. Consistent with previous results ( Fig. 1b ), Vγ6 gradually decreased in the thymus after birth and were scarce on day 17 ( Supplementary Fig. 4a ). Mature Vγ4 T cells were indeed increased over time and peaked at day 5 and then decreased, which is consistent with a previous study [13] . The ratios of matured Vγ4 versus Vγ6 were 1:5 at day 2, 1:1 at day 4, 4:1 at day 5. On day 17, almost no Vγ6 was found in the thymus ( Supplementary Fig. 4a ). After 8 weeks reconstitution, we examined γδT cell composition. Dermal γδT cells were fully reconstituted with thymocytes of days 2–5 mice ( Supplementary Fig. 4b ). Vγ6 T cells were predominant γδT cells in the skin although dermal Vγ4 T cells did increase using thymocytes of day 5 mice. However, this was not comparable with the ratio of matured Vγ4 versus Vγ6 in the thymus of day 5 mice (4:1). Both Vγ4 and Vγ6 were capable of producing IL-17 ( Supplementary Fig. 4c ). The unbalanced ratios of Vγ6 over Vγ4 were also shown in the lung but less striking in the peripheral blood, LN and spleen. Vγ4 and Vγ6 were almost at 1:1 ratio in the peripheral blood and LN using thymocytes from day 5 mice ( Supplementary Fig. 4d ). Dermal γδT cells were poorly reconstituted using thymocytes of day 17 mice, which predominantly constituted Vγ4. Taken together, these data suggest that thymic Vγ4 T cells may require an extrathymic environment to imprint their skin-homing properties, and that thymic Vγ6 T cells may be more competitive than Vγ4 for dermal γδT cell reconstitution. We also examined CCR6 expression on Vγ4 T cells since dermal γδT cells constitutively express CCR6 (ref. 4 ). Vγ4 T cells from neonatal thymus had almost no CCR6 expression, whereas Vγ6 T cells expressed an appreciable level of CCR6 ( Fig. 3d and Supplementary Fig. 3b ). In addition, 15% of Vγ4 T cells from BM expressed CCR6 ( Fig. 3d ), suggesting that BM Vγ4 T cells may have gained skin-homing receptor expression. Along this line, dermal Vγ4 T cells were significantly lower in CCR6-deficient mice but not in CCR10-deficient mice compared with those from WT mice ( Fig. 3e and Supplementary Fig. 3c ), although total dermal γδT cell frequency was not altered. In addition, the percentage of Vγ4 T cells in BM, LN or spleen was not significantly changed between WT and CCR6KO mice ( Fig. 3f and Supplementary Fig. 3d ), suggesting that CCR6 is not essential for Vγ4 T cell trafficking from fetal thymus to BM, LN or spleen but is critical for their homing to skin. Mice with predominate Vγ6 T cells develop skin inflammation We have previously shown that dermal γδT cells are critical in skin inflammation such as psoriasis [4] . Mice lacking Vγ4 IL-17T cells had significantly less epidermal thickening and neutrophil infiltration [13] . To determine whether Vγ6 T cells also have a role in skin inflammation, we used mice reconstituted with neonatal thymocytes plus BM cells, which predominantly express Vγ6 T cells, for IMQ topical treatment. Mice reconstituted with BM alone containing mainly Vγ4 were used as control. Consistent with the previous experiment ( Fig. 2a ), mice reconstituted with neonatal thymocytes plus BM cells had threefold more dermal γδT cells than mice reconstituted with BM alone ( Fig. 4a ). Despite lower frequency of dermal γδT cells in BM alone reconstituted mice, histological analysis showed similar levels of epidermal thickening (acanthosis) in both groups ( Fig. 4b ). Daily application of IMQ to the back skin significantly increased neutrophil infiltration and mRNA levels of IL-17 and IL-22 in both groups ( Fig. 4c ). In addition, the frequencies of IL-17-producing dermal γδT cells were also similar ( Fig. 4d ). To specifically demonstrate whether Vγ6 T cells are able to induce skin inflammation, we sorted Vγ6 from neonatal thymocytes and co-transferred with BM cells from TCRδ −/− mice into TCRδ −/− mice to eliminate any resident dermal γδT cells or γδT cells from BM cells ( Supplementary Fig. 5a ). The reconstituted mice expressed exclusive Vγ6 and developed severe skin inflammation upon IMQ topical treatment. The epidermal thickness and neutrophil infiltration were significantly increased as compared with TCRδ −/− mice ( Supplementary Fig. 5b,c ). In addition, mRNA levels of IL-17 and IL-22 were also significantly increased ( Supplementary Fig. 5d ). Taken together, these findings suggest that dermal Vγ6 T cells are pathogenic and are able to induce psoriasis-like dermatitis. However, Vγ4 T cells may be more prone to induce skin inflammation because reconstituted mice expressing Vγ4 develop similar magnitude of disease with significant fewer total dermal γδT cells. 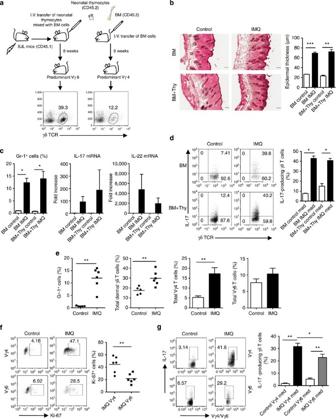Figure 4: Dermal Vγ6 T cells induce skin inflammation but dermal Vγ4 are preferentially expanded and are the major IL-17 producers. (a) BM cells or BM cells plus neonatal thymocytes (BM+Thy) from C57Bl/6 WT mice (CD45.2) were transplanted into lethally irradiated SJL mice (CD45.1,n=5). After 8 weeks of reconstitution, frequency of dermal γδT cells was detected by flow cytometry. Mice receiving BM cells alone predominantly reconstituted Vγ4, whereas mice receiving BM plus neonatal thymocytes predominantly reconstituted Vγ6. (b) Reconstituted mice were treated daily for 5 days with IMQ or control cream (control). Representative H&E-stained sections are shown and epidermal thickness were measured at day 5. Scale bar, 100 μm. Data are shown as mean±s.e.m. **P<0.01, ***P<0.001 (unpaired Student’st-test). (c) Percentage of CD45+Gr-1+cells after IMQ treatment was analysed by flow cytometry. IL-17 and IL-22 mRNA levels were measured by qPCR. Data are shown as mean±s.e.m. *P<0.05 (unpaired Student’st-test). (d) Intracellular IL-17 production by skin dermal γδT cells from IMQ-treated or control mice was determined by flow cytometry (without stimulation). Flow plots were gated on CD3+cells. Data are shown as mean±s.e.m. *P<0.05 (unpaired Student’st-test). (e) C57Bl/6 WT mice (n=5-6) were treated daily for 5 days with IMQ or control cream (control). Percentages of CD45+Gr-1+cells, total dermal γδT cells, dermal Vγ4 and Vγ6 cells were analysed by flow cytometry. Data are shown as mean±s.e.m. and are representative of two independent experiments with similar results. **P<0.01 (unpaired Student’st-test). (f,g) Ki-67 expression (f) and intracellular IL-17 production (g) by dermal Vγ4 and Vγ6 cells were determined by flow cytometry (without stimulation). Flow plots were gated on CD3intγδTCRintcells. Data are shown as mean±s.e.m. and are representative of two independent experiments with similar results. *P<0.05, **P<0.01 (unpaired Student’st-test). Figure 4: Dermal Vγ6 T cells induce skin inflammation but dermal Vγ4 are preferentially expanded and are the major IL-17 producers. ( a ) BM cells or BM cells plus neonatal thymocytes (BM+Thy) from C57Bl/6 WT mice (CD45.2) were transplanted into lethally irradiated SJL mice (CD45.1, n =5). After 8 weeks of reconstitution, frequency of dermal γδT cells was detected by flow cytometry. Mice receiving BM cells alone predominantly reconstituted Vγ4, whereas mice receiving BM plus neonatal thymocytes predominantly reconstituted Vγ6. ( b ) Reconstituted mice were treated daily for 5 days with IMQ or control cream (control). Representative H&E-stained sections are shown and epidermal thickness were measured at day 5. Scale bar, 100 μm. Data are shown as mean±s.e.m. ** P <0.01, *** P <0.001 (unpaired Student’s t -test). ( c ) Percentage of CD45 + Gr-1 + cells after IMQ treatment was analysed by flow cytometry. IL-17 and IL-22 mRNA levels were measured by qPCR. Data are shown as mean±s.e.m. * P <0.05 (unpaired Student’s t -test). ( d ) Intracellular IL-17 production by skin dermal γδT cells from IMQ-treated or control mice was determined by flow cytometry (without stimulation). Flow plots were gated on CD3 + cells. Data are shown as mean±s.e.m. * P <0.05 (unpaired Student’s t -test). ( e ) C57Bl/6 WT mice ( n =5-6) were treated daily for 5 days with IMQ or control cream (control). Percentages of CD45 + Gr-1 + cells, total dermal γδT cells, dermal Vγ4 and Vγ6 cells were analysed by flow cytometry. Data are shown as mean±s.e.m. and are representative of two independent experiments with similar results. ** P <0.01 (unpaired Student’s t -test). ( f , g ) Ki-67 expression ( f ) and intracellular IL-17 production ( g ) by dermal Vγ4 and Vγ6 cells were determined by flow cytometry (without stimulation). Flow plots were gated on CD3 int γδTCR int cells. Data are shown as mean±s.e.m. and are representative of two independent experiments with similar results. * P <0.05, ** P <0.01 (unpaired Student’s t -test). Full size image Normal naive mice have similar frequencies of dermal Vγ6 and Vγ4 T cells. We sought to determine whether dermal Vγ4 and Vγ6 T cells respond to IMQ differently in naive mice. As expected, mice applied with IMQ cream developed massive neutrophil infiltration ( Fig. 4e ). Total dermal γδT cells were also increased. Among them, dermal Vγ4 T cells were preferentially expanded as compared with Vγ6 ( Fig. 4e ). Ki-67 staining indicated that Vγ4 had significantly more proliferation than Vγ6 ( Fig. 4f ). To assess IL-17 production by dermal γδT cells ex vivo , skin tissues were digested and stained intracellularly for IL-17. Both Vγ4 and Vγ6 dermal T cells produced IL-17. However, Vγ4 T cells produced significantly more IL-17 than Vγ6 T cells ( Fig. 4g ). Thus, dermal Vγ4 T cells appear to have a more critical role compared with Vγ6 T cells in IMQ-induced psoriasis-like dermatitis. IL-23 and IL-1β differently regulate dermal Vγ4 and Vγ6 We reason that the differential responses to IMQ by dermal Vγ4 and Vγ6 T cells could be because of cytokine regulations, as the IMQ-induced psoriasis-like dermatitis model is dependent of the IL-23/IL-17 pathway [20] . To determine the role of IL-23 and IL-1β in the regulation of dermal γδT cells, whole-skin cells were labelled with carboxyfluorescein succinimidyl ester (CFSE) and stimulated with IL-23, IL-1β or IL-23 plus IL-1β. IL-23 alone or IL-1β alone was capable of driving dermal γδT cell proliferation ( Fig. 5a ). Combination of IL-23 and IL-1β did not significantly increase dermal γδT cell proliferation. In contrast, IL-17 production was largely induced upon IL-23 stimulation by both proliferated and unproliferated dermal γδT cells. IL-1β alone induced minimal IL-17 production. Combined IL-1β with IL-23 significantly enhanced IL-17 production. In addition, we found that either IL-23 or IL-1β was able to stimulate Vγ4 and Vγ6 proliferation. Strikingly, dermal Vγ4 T cells produced significantly more IL-17 than Vγ6 T cells upon IL-23 or IL-23 plus IL-1β stimulation ( Fig. 5b ). 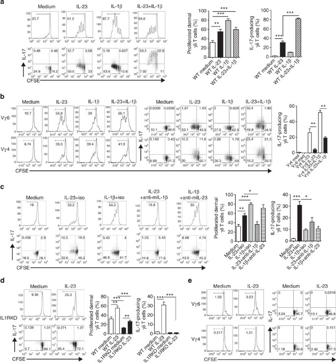Figure 5: IL-23 and IL-1β regulate dermal Vγ4 and Vγ6 γδT cell proliferation and IL-17 production. (a,b) Whole-skin cell suspensions were labelled with CFSE and then stimulated with IL-23, IL-1β or IL-23 plus IL-1β for 3 days. CFSE dilution and intracellular IL-17 production by dermal γδT cells (a) or dermal Vγ4 and Vγ6 γδT cells (b) were determined by flow cytometry. Flow plots gated on CD3intγδTCRintcells are representative of at least three independent experiments with similar results. Data are shown as mean±s.e.m. (n=10). **P<0.01, ***P<0.001 (unpaired Student’st-test). (c) Whole-skin cells suspensions were labelled with CFSE and then stimulated with IL-23, IL-1β, IL-23 plus anti-mouse IL-1β, IL-1β plus anti-mouse IL-23 or isotype control mAb in WT mice for 3 days. CFSE dilution and intracellular IL-17 production by dermal γδT cells were determined by flow cytometry. Flow plots gated on CD3intγδTCRintcells are representative of at least three independent experiments with similar results. Summarized data (n=8–9) are shown as mean±s.e.m. *P<0.05, **P<0.01, ***P<0.001 (unpaired Student’st-test). (d,e) Whole-skin cells suspensions from IL-1RI KO mice labelled with CFSE were stimulated with IL-23 for 3 days. CFSE dilution and intracellular IL-17 production by dermal γδT cells (d) or dermal Vγ4 and Vγ6 γδT cells (e) were determined by flow cytometry. Flow plots gated on CD3intγδTCRintcells are representative of at least three independent experiments with similar results. Data are shown as mean±s.e.m. (n=8-9). **P<0.01, ***P<0.001 (unpaired Student’st-test). Figure 5: IL-23 and IL-1β regulate dermal Vγ4 and Vγ6 γδT cell proliferation and IL-17 production. ( a , b ) Whole-skin cell suspensions were labelled with CFSE and then stimulated with IL-23, IL-1β or IL-23 plus IL-1β for 3 days. CFSE dilution and intracellular IL-17 production by dermal γδT cells ( a ) or dermal Vγ4 and Vγ6 γδT cells ( b ) were determined by flow cytometry. Flow plots gated on CD3 int γδTCR int cells are representative of at least three independent experiments with similar results. Data are shown as mean±s.e.m. ( n =10). ** P <0.01, *** P <0.001 (unpaired Student’s t -test). ( c ) Whole-skin cells suspensions were labelled with CFSE and then stimulated with IL-23, IL-1β, IL-23 plus anti-mouse IL-1β, IL-1β plus anti-mouse IL-23 or isotype control mAb in WT mice for 3 days. CFSE dilution and intracellular IL-17 production by dermal γδT cells were determined by flow cytometry. Flow plots gated on CD3 int γδTCR int cells are representative of at least three independent experiments with similar results. Summarized data ( n =8–9) are shown as mean±s.e.m. * P <0.05, ** P <0.01, *** P <0.001 (unpaired Student’s t -test). ( d , e ) Whole-skin cells suspensions from IL-1RI KO mice labelled with CFSE were stimulated with IL-23 for 3 days. CFSE dilution and intracellular IL-17 production by dermal γδT cells ( d ) or dermal Vγ4 and Vγ6 γδT cells ( e ) were determined by flow cytometry. Flow plots gated on CD3 int γδTCR int cells are representative of at least three independent experiments with similar results. Data are shown as mean±s.e.m. ( n =8-9). ** P <0.01, *** P <0.001 (unpaired Student’s t -test). Full size image Whole-skin cells contain endogenous IL-1β presumably produced by skin resident cells [21] , [22] . We next determined whether the proliferation of dermal γδT cells induced by IL-23 is dependent on IL-1β and conversely whether IL-1β-induced γδT cell proliferation is dependent on IL-23. Using neutralizing monoclonal antibodies (mAbs) against IL-23 and IL-1β and corresponding isotype control mAbs, we found that the proliferation and IL-17 production by dermal γδT cells in response to IL-23 stimulation were significantly decreased when blocking endogenous IL-1β ( Fig. 5c ). In contrast, IL-1β-induced dermal γδT cell proliferation and IL-17 production were not significantly influenced by IL-23 ( Fig. 5c ). Thus, IL-1β appears to be critical in both dermal γδT cell proliferation and IL-17 production induced by IL-23. We next used IL-1RI knockout (KO) mice to examine the regulatory role of IL-1β in dermal γδT cells. There was a significant lower basal level of proliferated dermal γδT cells in IL-1RI KO mice compared with WT mice ( Fig. 5d ). Dermal γδT cell proliferation was still observed upon IL-23 stimulation in IL-1RI KO mice, although the overall level was significantly lower than WT mice ( Fig.5d ). IL-17 production was completely abrogated in IL-1RI KO mice. Further dermal γδT cell subset studies indicated that dermal Vγ6 but not Vγ4 T cells had IL-23-induced proliferation independent of IL-1β signalling ( Fig. 5e ). However, IL-17 production by dermal Vγ4 and Vγ6 both required IL-1R signalling. Thus, IL-23-induced dermal Vγ6 T-cell proliferation has both IL-1β-dependent and -independent pathways. However, IL-1β signalling is essential for IL-23-induced dermal γδT cell IL-17 production. IL-1β stimulates KCs for chemokine production IL-1β has been identified as a key inflammatory cytokine in the pathogenesis of cutaneous inflammation including psoriasis [23] . Elevated IL-1β levels were reported in psoriatic skin lesions [24] . To further delineate the role of IL-1β on KC activation, we treated primary murine KC cells with IL-1β, and found that mRNA levels of chemokines including CCL2, CCL5, CCL20, CXCL9 and CXCL10 were increased ( Fig. 6a ), suggesting that IL-1β may modulate dermal γδT cell trafficking. CCL20-CCR6 axis has been implicated in dermal γδT cell trafficking and psoriasis pathogenesis [25] , [26] . To investigate whether γδT cells could migrate from peripheral lymphoid organs into dermis in addition to already established resident γδT cells, we sorted γδT cells from spleen and LN and then adoptively transferred them into SJL mice. As depicted in Fig. 6b , γδT cells migrated into dermis and expressed CCR6. γδT cells from CCR6-deficient mice had significantly lower frequency in dermis, suggesting that CCR6 is critical in peripheral γδT cell trafficking into skin. In addition, no difference was observed in other anatomical sites ( Fig. 6b ). 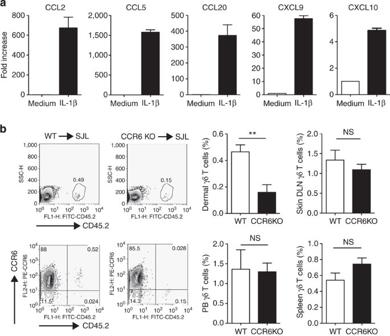Figure 6: CCR6 is essential for γδT cell trafficking from periphery to dermis. (a) Primary murine KC were stimulated with IL-1β for 6 h. CCL2, CCL5, CCL20, CXCL9 and CXCL10 mRNA levels were measured by qPCR. The figure shows fold changes normalized for β-MG mRNA versus medium alone. Data are shown as mean±s.e.m. (b) Sorted γδT cells from spleen and LN from C57Bl/6 WT mice or CCR6KO mice were adoptively transferred into SJL mice (n=4). After 5–7 days, cells from skin, peripheral blood, LN and spleen were stained with CD3, γδ TCR and CCR6. Frequency of total γδT cells and CCR6+γδT cells from donor (CD45.2) were determined by flow cytometry. Flow plots were gated on skin CD3intγδTCRintcells. Data are shown as mean±s.e.m. **P<0.01, NS, not significant (unpaired Student’st-test). Figure 6: CCR6 is essential for γδT cell trafficking from periphery to dermis. ( a ) Primary murine KC were stimulated with IL-1β for 6 h. CCL2, CCL5, CCL20, CXCL9 and CXCL10 mRNA levels were measured by qPCR. The figure shows fold changes normalized for β-MG mRNA versus medium alone. Data are shown as mean±s.e.m. ( b ) Sorted γδT cells from spleen and LN from C57Bl/6 WT mice or CCR6KO mice were adoptively transferred into SJL mice ( n =4). After 5–7 days, cells from skin, peripheral blood, LN and spleen were stained with CD3, γδ TCR and CCR6. Frequency of total γδT cells and CCR6 + γδT cells from donor (CD45.2) were determined by flow cytometry. Flow plots were gated on skin CD3 int γδTCR int cells. Data are shown as mean±s.e.m. ** P <0.01, NS, not significant (unpaired Student’s t -test). Full size image IL-1R signalling is critical in skin inflammation We next examined whether IL-1β is involved in the skin inflammation such as psoriasis. As previously reported, both IL-23 dermal injection and IMQ induce human psoriasis-like skin inflammation and pathology [20] , [27] . The epidermal hyperplasia and neutrophil infiltration induced by IMQ or IL-23 were markedly decreased in IL-1RI KO mice compared with WT mice ( Fig. 7a and Supplementary Fig. 6a ). In addition, the mRNA levels of IL-17 and IL-22 were also significantly decreased in IL-1RI KO mice ( Fig. 7b and Supplementary Fig. 6b ). Further analysis of IL-17-producing dermal γδT cells from treated and untreated skin tissues indicated that the basal levels of IL-17-producing dermal γδT cells were significantly lower in IL-1R KO mice compared with those in WT mice ( Fig. 7c and Supplementary Fig. 6c ). Upon IL-23 or IMQ treatment, dermal γδT cells secreted large amounts of IL-17 in WT mice, and IL-17 levels were significantly more in WT mice as compared with IL-1RI KO mice ( Fig. 7c and Supplementary Fig. 6c ). Taken together, these data suggest that IL-1RI expression is critical in both IL-23 and IMQ-induced skin inflammation and acanthosis. 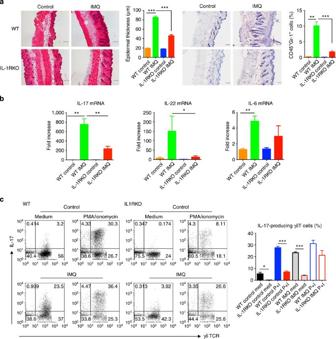Figure 7: IL-1R signalling is essential for IMQ-induced skin inflammation and acanthosis. (a) C57Bl/6 WT and IL-1RI KO mice (n=6–8) were treated daily for 5 days with IMQ or control cream (control). Representative H&E-stained sections and frozen sections stained with Gr-1 are shown. Gr-1 positive cells are brown. Skin tissues were also stained with CD45 and Gr-1 assessed by flow cytometry. Epidermal thickness and percentage of CD45+Gr-1+cells were measured at day 5. Scale bar, 100 μm. Data are shown as mean±s.e.m. **P<0.01, ***P<0.001 (unpaired Student’st-test). (b) IL-17, IL-22 and IL-6 mRNA levels were measured by qPCR. The figure shows fold changes normalized for β-MG mRNA versus control skin from WT mice. Data are shown as mean±s.e.m. *P<0.05, **P<0.01 (unpaired Student’st-test). (c) Intracellular IL-17 production by dermal γδT cells with or without PMA plus ionomycin stimulation was determined by flow cytometry. Flow plots were gated on CD3+cells. Data are shown as mean±s.e.m. *P<0.05, ***P<0.001 (unpaired Student’st-test). Figure 7: IL-1R signalling is essential for IMQ-induced skin inflammation and acanthosis. ( a ) C57Bl/6 WT and IL-1RI KO mice ( n =6–8) were treated daily for 5 days with IMQ or control cream (control). Representative H&E-stained sections and frozen sections stained with Gr-1 are shown. Gr-1 positive cells are brown. Skin tissues were also stained with CD45 and Gr-1 assessed by flow cytometry. Epidermal thickness and percentage of CD45 + Gr-1 + cells were measured at day 5. Scale bar, 100 μm. Data are shown as mean±s.e.m. ** P <0.01, *** P <0.001 (unpaired Student’s t -test). ( b ) IL-17, IL-22 and IL-6 mRNA levels were measured by qPCR. The figure shows fold changes normalized for β-MG mRNA versus control skin from WT mice. Data are shown as mean±s.e.m. * P <0.05, ** P <0.01 (unpaired Student’s t -test). ( c ) Intracellular IL-17 production by dermal γδT cells with or without PMA plus ionomycin stimulation was determined by flow cytometry. Flow plots were gated on CD3 + cells. Data are shown as mean±s.e.m. * P <0.05, *** P <0.001 (unpaired Student’s t -test). Full size image In this study, we examine dermal γδT cell development and find that these cells are scarce on E20 and neonatal pups but become obvious at day 3. They predominately express Vγ6 TCR, suggesting that Vγ6 T cells are bona fide resident dermal γδT cells. After birth, dermal γδT cells undergo haemostatic proliferation with diversified TCR repertoire. Vγ4 T cells gradually increase over time in the dermis. This striking ontogeny profile may imply differential functions for dermal γδT cells with a distinct TCR repertoire. This is also in sharp contrast with lung γδT cells, which appear on E20 and maintain similar ratios of Vγ4 and Vγ6 in different ages of mice. Interestingly, conventional αβT cells occur in a significantly delayed fashion, suggesting that one of the primary contributions of dermal γδT cells is neonatal skin protection. Previous studies suggest that DETCs or innate-like CD27 − IL-17-producing cells cannot be generated from the BM [28] . However, it is not definitive whether dermal γδT cells can be reconstituted by BM cells [5] , [6] , [11] , [13] . Our study clearly shows that dermal γδT cells can be reconstituted from the BM, although thymus is absolutely required. This suggests that the precursors of dermal γδT cells in the BM are probably re-circulated from the thymus. The precursors of dermal γδT cells in the BM contain mainly Vγ4 and Vγ1 but not Vγ6. As shown in our study, Vγ6 T cells can be directly reconstituted from fetal thymus. It appears that this extra detour for thymic Vγ4 T cells is to gain skin-homing properties. It is possible that transferred neonatal thymic Vγ4 T cells may require a longer time for skin seeding as compared with adult BM Vγ4. Using thymocytes from different ages of mice, we showed that matured Vγ4 T cells are significantly increased and are more than matured Vγ6 T cells in the thymus of day 5 mice. However, Vγ6 T cells are still the predominant dermal γδT cells in the reconstituted mice. This is different from γδT cell composition in the peripheral blood and LN, suggesting that thymic Vγ4 T cells need extrathymic environment for imprinting their skin-homing properties, such as gaining an activated status or CCR6 expression that enables them home to the skin or sites of inflammation. It also suggests that thymic Vγ6 T cells may be more competitive than Vγ4 for dermal γδT cell reconstitution. Although it is unclear which factor(s) stimulates thymic egressed Vγ4 T cells for imprinting of their skin-homing capability, it is conceivable that Ag stimulation may be one of driving forces for their maturation and functional competency. Indeed, a recent study showed that γδT cells recognize a microbial-encoded B-cell Ag for activation and IL-17 production [29] . These distinct developmental requirements between dermal Vγ4 and Vγ6 T cells are also supported by two recent studies showing their differential transcription factors for programming such as SOX4 and SOX13, respectively [13] , [14] . It is thus proposed that dermal γδT cells contain bona fide resident Vγ6 T cells that are non-migratory, mature γδT cells with IL-17-producing ability and are the major force in the network of neonatal skin immunosurveillance. In contrast, dermal Vγ4 T cells, which require extrathymic environment for imprinting their skin-homing properties, are probably migratory and the inducible IL-17-producing cells. Vγ4 T cells can be Ag-specific and produce large amounts of IL-17 in the presence of TCR engagement, thus perpetuating the IL-17 response in inflammation [30] . Dermal Vγ4 and Vγ6 T cells also use differential chemokine receptors for their skin homing. Deficiency of CCR6 or CCR10 alone does not significantly alter dermal Vγ6 T-cell skin migration. However, dermal Vγ4 T cells are significantly lower in CCR6-deficient mice but not in CCR10-deficient mice. CCR6 is critical for Vγ4 T cells in the BM homing to skin but not essential for Vγ4 thymic egress, as frequencies of Vγ4 T cells in the BM of WT or CCR6 KO mice are similar. Although Vγ4 and Vγ6 dermal γδT cells have differential developmental requirement, it appears that both subsets are functional competent in terms of IL-17 production and induction of psoriasis-like skin inflammation. This is different from previous studies using Sox13-deficient mice or Sox13 spontaneous mutant mice [13] , [14] . The discrepancy may arise from the overall frequency of dermal γδT cells. IL-17-producing Vγ4 T cells are selectively deficient in Sox13-mutated mice [13] and T-Sox4-deficient mice [14] , thereby leading to reduced skin inflammation. In our study, mice transplanted with fetal thymus or sorted Vγ6 from neonatal thymocytes have exclusively IL-17-producing Vγ6 T cells with the overall frequency similar as WT mice and develop severe skin inflammation upon IMQ treatment. Thus, it appears that the different results could be in part owing to the quantity of total IL-17-producing γδT cells in dermis. However, in naive mice where both dermal Vγ4 and Vγ6 T cells exist, Vγ4 T cells are preferentially expanded and are the major IL-17 producers upon IMQ topical treatment, suggesting that a peripheral regulation programme could be different for dermal Vγ4 and Vγ6 T cells. Although γδT cells are considered as pre-committed functional competent cells, dermal γδT cells are subject to peripheral regulation. We found that IL-1β and IL-23 are both capable of stimulating Vγ4 and Vγ6 T-cell proliferation. IL-23-stimulated dermal γδT cell proliferation is largely driven by IL-1β signalling but also has a IL-1 independent pathway, mainly with Vγ6. It is possible that endogenous levels of IL-18 could effect in conjunction with IL-23 to stimulate minimal dermal γδT cell proliferation in the absence of IL-1β, as IL-18 is critical in human γδT cell expansion and is independent of IL-1R signalling [31] . We also found that dermal Vγ4 cells are the major IL-17 producer as compared with dermal Vγ6 upon IL-23 or IL-23 plus IL-1β stimulation. This in vitro study is consistent with in vivo IMQ-induced psoriasis model in naive mice where IL-17-producing Vγ4 T cells are significantly expanded. However, the molecular mechanism accounting for these differences between Vγ4 and Vγ6 is not presently known. Both dermal Vγ4 and Vγ6 T cells are CD44 hi CD62L lo CD24 lo CD27 − and constitutively express CCR6 and RORγt ( Supplementary Fig. 7 ). They do not express NK1.1 as most NK1.1 + γδT cells produce IFN-γ [32] . IL-23R expression level is also low in both subsets, which may be related to their activation status [33] . Previous studies also identify scavenger receptor SCART2 is uniquely expressed in IL-17-producing γδT cells [15] . Nevertheless, we found that IL-1β is essential in both Vγ4 and Vγ6 T cell IL-17 production. Thus, IL-1β is not only critical in regulating dermal γδT cell expansion under inflammatory conditions but also is essential for dermal γδT cell effector function. IL-1β also stimulates KC to secrete many chemokines including CCR6 ligand CCL20. Since CCL20 expression is higher in skin inflammation such as psoriasis [34] , this raises the possibility that IL-1β signalling may be involved in dermal γδT cell trafficking via chemokine secretion. We show that peripheral γδT cells can be trafficked into the skin in a CCR6-dependent manner. Previous studies show that only CCR6 + γδT cells produce IL-17 (ref. 32 ). CCR6 + γδT cells are also found in the cerebrospinal fluid in multiple sclerosis patients [35] and in other inflammatory conditions [36] . However, CCR6 may be specific for Vγ4 T-cell peripheral trafficking into skin because Vγ6 T cells are minimal in draining lymph nodes (DLNs). This corroborates with a recent study showing two ways of Vγ4 dermal γδT cell migration from skin to draining LNs and back to inflamed skin [13] . This may also be related to previous studies showing that CCR6 KO mice have decreased skin inflammation in a murine psoriasis model [25] , [37] , [38] . IL-1β has also been demonstrated to have an important role in the course of cutaneous inflammation such as psoriasis [39] , [40] . Psoriatic lesions are found to have increased IL-1β mRNA expression and caspase-1 activation, which is responsible for cleaving the inactive precursor of IL-1β into active form [24] , [41] . Indeed, mice with excessive IL-1β expression or the lack of IL-1R antagonist ( Il1rn −/− ) develop a psoriasis-like skin inflammation [42] , [43] , [44] . In contrast, neutrophil infiltration and epidermal thickness are significantly decreased in IL-1RI-deficient mice. This is consistent with the overall significantly decreased IL-17-producing γδT cells in the skin. In addition, mRNA levels of IL-17 and IL-22 in IL-1RI KO mice were significantly lower than WT mice. Although there is still controversy over the treatment of psoriasis patients with IL-1R antagonist, a promising therapeutic efficacy of targeting IL-1 pathway has been reported from a small clinical trial, indicating the importance of IL-1 signalling in the development of human psoriasis [45] , [46] . Mice C57Bl/6 WT, B6.SJLWT, TCRd −/− , CCR6 −/− and Il1r1 −/− on C57Bl/6 background (female, 6–8 weeks old) were purchased from Jackson Laboratory. Nude mice (female, 6–8 weeks old) on C57Bl/6 background were purchased from Taconic. CCR10 KO mice were described previously [19] . All animals were housed and treated in accordance with institutional guidelines and approved by the Institutional Animal Care and Use Committee (IACUC) at the University of Louisville. Tissue preparation and cell stimulation Whole-skin cells were prepared from mouse back skin [4] . In brief, skin tissues were digested with a buffer containing collagenase IV, hyaluronidase and DNase I. Skin cells were labelled with CFSE and stimulated with rIL- 23 (1 ng ml −1 , eBioscience), rIL-1β (1 ng ml −1 , eBioscience) or rIL-23 plus rIL-1β for 3 days. Cell proliferation and intracellular IL-17 were measured by flow cytometry. For blocking experiment, neutralizing mAbs for IL-1β (2 μg ml −1 , eBioscience), IL-23 (12.5 μg ml −1 , eBioscience) or matched isotype control mAbs were added. In addition, primary mouse KCs (Cellntec) were stimulated with IL-1β for 6 h and RNA were extracted for analysis of chemokine expression by real-time quantitative PCR (qPCR). For γδT cell development study, skin, thymus and BM were taken from pups before (E18 or E20) or after birth. Flow cytometry analysis and intracellular cytokine staining Fluorochrome-labelled mAbs including mouse γδTCR (GL3, 1:100), Vγ4 (UC3-10A6, 1:500), Vγ1 (2.11, 1:500), CD24 (M1/69, 1:500), CD27 (LG.3A10, 1:500), CD62L (MEL-14, 1:500) and IL-17A (TC11-18H10.1, 1:500, Biolegend), CD44 (IM7, 1:200), RORγt (AFKJS-9, 1:200), and Ki-67 (SolA15, 1:200, eBioscience), IL-23R (753317, 1:10) and CCR6 (140706, 1:50, R&D Systems) were used. Anti-mouse Vγ6 (17D1, 1:500) was kindly provided by Dr. Tigelaar (Department of Dermatology, Yale University). For intracellular cytokine staining, cells were first blocked with anti-CD16/32 and then stained with different cell surface antibodies (Abs). Cells were then fixed, permeabilized and stained intracellularly for IL-17, RORγt or Ki-67. The relevant isotype control mAbs were also used. Samples were harvested with BD FACS Calibur or Canto (Becton Dickinson, San Jose, CA, USA) and analysed with FlowJo software (TreeStar). BM chimeras The BM chimeras were generated as previously reported [5] . In brief, recipient mice were lethally irradiated with 950 cGy and then were intravenously transferred with 5-10 × 10 6 thymocytes. After 24 h, the recipient mice received 5–10 × 10 6 BM cells. In some experiments, the lethally irradiated WT, nude or TCRd −/− mice were transferred with BM cells alone. In addition, sorted Vγ4 or Vγ6 γδT cells from C57Bl/6 neonatal thymocytes mixed with BM cells from SJL mice were transferred into irradiated TCRd −/− mice. In some experiments, sorted Vγ6 cells from neonatal thymocytes plus BM cells from TCRd −/− mice were transferred into irradiated TCRd −/− mice. Neonatal thymocytes used in all experiments were taken from pups born within 48 h. All chimeric mice were allowed to reconstitute for at least 8 weeks before use in experiments. Peripheral γδT cells trafficking γδT cells were sorted from LN and spleens from C57Bl/6 or CCR6 −/− mice and then intravenously transferred to SJL mice. After 5–7 days, recipient mice were killed. Peripheral blood, skin, LN and spleen samples were collected for further analysis of the expression of γδT cells from donor by flow cytometry. Establishment of psoriasis-like mouse models IL-23-induced psoriasis-like mouse model was established as previously described [27] . In brief, IL-23 (1 μg) or vehicle control was daily intradermally injected on the back skin of WT or Il1r1 −/− mice for 4 days. For IMQ-induced psoriasis-like model [20] , WT or Il1r1 −/− mice were applied daily with IMQ cream (5%; Aldara; 3M Pharmaceuticals) for 5 consecutive days. In some experiments, BM chimera mice were also applied with IMQ. Mice were killed and the skin samples were embedded and frozen in (optimal cutting temperature (OCT) for hematoxylin and eosin (H&E) and immunohistochemistry (IHC) staining. Skin samples were also excised in TRIzol (Invitrogen) for RNA extraction. Skin cell suspensions were stained for Gr-1 expression and IL-17 production. Skin histology and IHC staining Skin sections were stained with H&E and the epidermal thickness was determined by measuring the average interfollicular distance under the microscope in a blinded manner. For IHC staining, skin cryosections were fixed, blocked and stained with rat-anti-mouse Gr-1 mAb (1:50) followed by goat-anti-rat IgG secondary Ab (1:200, Southern Biotech) [4] . Slides were developed with 3-amino-9-ethylcarbazole substrate solution (Vector Laboratories) and counterstained with hematoxylin. Images were acquired at × 200 magnification using Aperio ScanScope digital scanners. RNA extraction and real-time qPCR RNAs were isolated using a Qiagen RNeasy kit. After reverse transcription into cDNA, qPCR was performed on Bio-Rad MyiQ single colour real time (RT)–PCR detection system using SYBR Green Supermix (Bio-Rad) and gene-specific primers were listed as follows: all chemokines (Real Time Primers, LLC, Elkins Park, PA, USA); IL-17A (Mm_Il17a_SG, Qiagen); IL-22: 5′-ATACATCGTCAACCGCACCTTT-3′ (forward), 5′-AgCCGGACATCTGTGTTGTTAT-3′ (reverse); IL-6: 5′-GAGAAAAGAGTTCAATGGC-3′ (forward), 5′-CCA GTT TGG TAG CAT CCA TCA T-3′ (reverse). We normalized gene expression level to β-2 microglobulin (β-MG) housekeeping gene and represented data as fold differences by the 2 −ΔΔCt method, where Δ C t=Ct target gene − C t β-MG and ΔΔ C t=Δ C t induced −Δ C t reference . Statistical analysis All quantitative data are shown as mean±s.e.m. unless otherwise indicated. All samples were compared using two-tailed, unpaired Student’s t -test. A P value <0.05 was considered significant. Statistical analysis was performed with GraphPad Prism software. How to cite this article: Cai, Y. et al . Differential developmental requirement and peripheral regulation for dermal Vγ4 and Vγ6T17 cells in health and inflammation. Nat. Commun. 5:3986 doi: 10.1038/ncomms4986 (2014).